Carbonate-hosted methanotrophy represents an unrecognized methane sink in the deep sea The atmospheric flux of methane from the oceans is largely mitigated through microbially mediated sulphate-coupled methane oxidation, resulting in the precipitation of authigenic carbonates. Deep-sea carbonates are common around active and palaeo-methane seepage, and have primarily been viewed as passive recorders of methane oxidation; their role as active and unique microbial habitats capable of continued methane consumption has not been examined. Here we show that seep-associated carbonates harbour active microbial communities, serving as dynamic methane sinks. Microbial aggregate abundance within the carbonate interior exceeds that of seep sediments, and molecular diversity surveys reveal methanotrophic communities within protolithic nodules and well-lithified carbonate pavements. Aggregations of microbial cells within the carbonate matrix actively oxidize methane as indicated by stable isotope FISH–nanoSIMS experiments and 14 CH 4 radiotracer rate measurements. Carbonate-hosted methanotrophy extends the known ecological niche of these important methane consumers and represents a previously unrecognized methane sink that warrants consideration in global methane budgets. Methane has played an important role in global climate change in the past and remains the fourth most significant contributor to greenhouse forcing [1] , motivating the characterization of methane’s sources, sinks and fluxes. Biologically mediated, sulphate-coupled anaerobic oxidation of methane (AOM) is the dominant sink for methane in the oceans, consuming an estimated 382 Tg CH 4 per year in seafloor sediments, a quantity equivalent to ~88% of the methane released from subsurface reservoirs [2] . Microbiological study of AOM at methane seeps has focused almost exclusively on sediment-based habitats, where the most energetically favourable geochemical horizon, the sulphate–methane transition zone, typically occurs in the top several centimetres [3] . However, sediment accounts for only a portion of the seafloor cover at methane seep structures: based on sidescan sonar imagery and seafloor video observations, substantial portions of actively seeping areas are capped by carbonate rock precipitate [4] , [5] , [6] , [7] . The presence and potential activity of extant microbial communities within these carbonate rocks and their impact on global methane dynamics have so far been unexplored. In anoxic sediments at methane seeps, advection-driven methane-rich fluids come into contact with sulphate-rich seawater [8] . At these sites, biological AOM is mediated through an enigmatic metabolic partnership involving anaerobic methanotrophic (ANME) archaea and sulphur-metabolizing deltaproteobacteria that operates at a low predicted Gibbs energy yield [9] , [10] , [11] . The overall reaction of combined AOM and sulphate reduction increases alkalinity, promoting the precipitation of authigenic carbonate [12] . An estimated 14% of biologically oxidized methane at active seep settings precipitates in this manner [13] , leading to a range of carbonate minerals [14] . The resulting precipitation products may vary in size, ranging from microcrystals [15] to extensive structures of pavements, slabs and mounds produced by upward growth (known as chemoherms) or post-formation winnowing [14] , [16] , [17] . Carbonate volumes have been estimated for a few regions of active seepage and may exceed a million cubic metres at areas such as the Costa Rica margin [4] , Hydrate Ridge [6] and the Chilean subduction zone [5] , suggesting that these methane-derived structures have the potential to serve as a significant habitat within the seep ecosystem. The association of ANME microbial biomass with authigenic carbonates has been previously discussed in specialized environments. Most prominently, methane-fueled ‘reefs’ composed of porous carbonates and thick mats of ANME archaea and sulphate-reducing bacteria (SRB) were discovered at sites of vigorous methane venting in the euxinic bottom waters of the Black Sea [18] . Organic geochemical analysis of microbial mats within centimetre-scale void spaces within carbonate chemoherms from the Black Sea were found to contain lipids indicative of ANME and SRB; it was proposed that these carbonate structures formed through AOM-mediated carbonate precipitation in the sediment and, after sufficient accumulation, expanded into the overlying anoxic water column [19] . Although the discovery of the Black Sea AOM ecosystem has expanded our view of anaerobic methanotrophy and carbonate precipitation, the unique geochemical setting of this euxinic basin makes it difficult to extrapolate associated findings to the more globally relevant carbonate precipitation associated with AOM along continental margins. At such locations, carbonate slabs and pavements range from outcrops of vuggy, highly porous rock to lower-permeability massive structures [6] , [16] . Sr-isotope data and the presence of carbonate precipitation products favoured under high-bicarbonate, low-sulphate conditions suggest that carbonate is largely precipitated within the sediment, and is subsequently exposed through uplift and/or erosion [16] . There is no large-scale visible surficial manifestation of ANME/SRB biomass, as observed in the Black Sea [18] , and the potential for carbonate-associated methanotrophic activity by extant endoliths (organisms living within the pore spaces of rocks) has not been examined. In select seep settings along continental margins and submarine mud volcanoes, archaeal 16S ribosomal RNA gene surveys and lipid biomarker analyses of carbonate crusts provided evidence of methanotrophic microbial biosignatures [20] . Within porous Hydrate Ridge chemoherms experiencing focused fluid flow, isotopic links between AOM and carbonates were reported, as were putative fossilized microbial filaments [6] . In both cases, the potential occurrence of intact, viable microorganisms and active methane oxidation within the carbonate matrix was not determined. The conditions in which microbial AOM has been suggested to occur alongside carbonate precipitation products [18] , [19] , [20] , [21] represent an end-member of potential endolithic habitats: settings with high connectivity to metabolic reactants (for example, methane and sulphate) and seemingly minor physicochemical or energetic obstacles to sulphate-dependent AOM. Well-lithified massive carbonate rocks that pave substantial areas of the seafloor associated with present and past methane seepage, as well as those precipitates found in areas of low seepage activity, represent unique endolithic habitats more constrained by permeability limitations and/or methane supply; the potential of methanotrophic activity in such settings warrants investigation. When subseafloor environments are considered, well-lithified rock constitutes the volumetrically dominant physical substrate at seep-associated mounds [4] , [5] , [6] , [14] . Although some endolithic organisms appear to gain nutrients from their host rock [22] , the self-sealing effect of microbially accelerated authigenic carbonate formation implies that the supply of energy and nutrients may be limited in the seep-associated endolithic habitat, offering a valuable comparison with the better-studied sediment-hosted methane seep communities. Carbonate mounds such as those at Hydrate Ridge, Oregon, are made up of several different lithologies, the most prominent being grey micrite-cemented massive carbonates and white aragonitic breccias that exhibit a range of porosities [6] , [14] . These rocks form extensive cohesive structures at seep sites, often extending hundreds of metres beneath the seafloor [5] , [23] . Endoliths are probably pervasive within rocks at the Earth’s surface [22] and have been observed within basaltic oceanic crust on the seafloor [24] and in deep subseafloor samples [25] . Endoliths are more formally divided into chasmo-, crypto- and eu-endoliths depending on their mode of rock colonization [26] ; the microorganisms referred to in this study with the more general term ‘endolith’ belong to a separate subset of organisms that precipitate authigenic rock around them in a process of gradual self-entombment. Geobiological studies that have examined authigenic carbonate mounds have primarily pursued biomarker characterization rather than modern endolithic activity. 13 C-depleted lipids such as crocetane and archaeol at Aleutian margin seeps [27] , lipids and ANME 16S rRNA genes at Gulf of Cadiz structures [28] , and an ANME-2-derived extended sn-2-hydroxyarchaeol found in multiple seep carbonate mounds [29] are all suggestive of methanotrophic archaeal involvement, but offer limited insight on contemporary metabolic activity. The presence of biomarkers within mounds is often used forensically in an effort to reconstruct antecedent microbial communities and past conditions of carbonate precipitation [30] ; such studies have offered evidence of AOM and methanogenesis in association with authigenic carbonates during and potentially after their formation [31] . The suggestion of microbial involvement with carbonate crust formation [20] , predicated on the detection of low-abundance ANME 16S rRNA gene sequences and 13 C-depleted archaeal lipids, challenged the interpretation of carbonate precipitation products as exclusively fossil deposits. However, the viability of the microbial community and sustained endolithic AOM activity within the authigenic carbonate matrix was not demonstrated. Seafloor and sediment-hosted authigenic carbonates have not historically been considered to be dynamic living ecosystems whose biological activity has a significant impact on seafloor methane fluxes; the findings presented here suggest that is precisely the case. We use molecular diversity surveys and fluorescence in situ hybridization (FISH) to demonstrate that methane-derived authigenic carbonates, including sediment-hosted protolithic nodules and exhumed carbonate rocks from both actively venting and low methane flux environments, are viable habitats for abundant methanotrophic microorganisms. Stable isotope analyses of carbonate-associated microorganisms by nanoscale secondary ion mass spectrometry (nanoSIMS) and 14 CH 4 radiotracer studies confirmed aerobic methanotrophic and ANME activity, revealing seafloor carbonate habitats as important, previously unrecognized methane sinks. 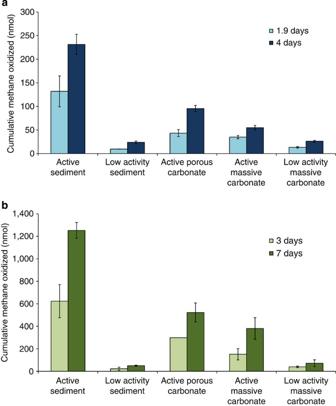Figure 1: Methane oxidation rates derived from14CH4radiotracer experiments. Rates under (a) oxic and (b) anoxic conditions are shown, using active sediment (A.Sed-5128), low-activity sediment (L.Sed-5043) and intact pieces of active porous carbonate (A.Carb-5305), active massive carbonate (A.Carb-5152) and low-activity massive carbonate (L.Carb-5028) from Hydrate Ridge. Each bar represents nmol methane oxidized at a particular time point, with values from killed control experiments subtracted; error bars show s.e. for triplicate incubations (the 1.9-day aerobic low-activity sediment and 3-day anaerobic active porous carbonate data points represent only one replicate). Characterizing the endolithic habitat Twenty-four samples were collected for study from methane seep sites at Hydrate Ridge, Eel River Basin and the Costa Rica margin ( Supplementary Table 1 and Supplementary Figs 1 and 2 ). 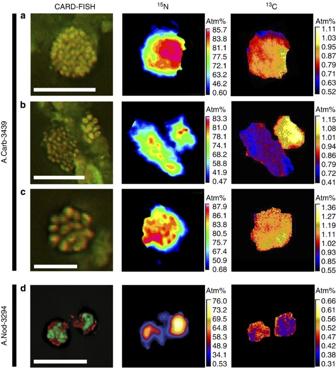Figure 2: Anabolic incorporation of isotopically labelled substrate by endolithic microbial aggregates. Paired CARD-FISH and nanoSIMS results of samples A.Carb-3439 (a–c) and A.Nod-3294 (d) are provided. A.Carb-3439 was incubated at 4 °C for 27 months under anoxic conditions with 2 mM15NH4Cl and 1.48 mM CH4(50%13CH4); A.Nod-3294 was incubated at 4 °C for 9 months under anoxic conditions with 1 mM15NH4and 1.12 mM12CH4. In A.Carb-3439 CARD-FISH images, red signal indicates Arch 915 hybridization and green indicates DSS 658 hybridization; the colours are reversed for A.Nod-3294 hybridizations.15N and13C atom % nanoSIMS images are derived from15N12C−/14N12C−and13C−/12C−ion count ratios, respectively, and represent mean values from multiple planes of analysis. Scale bars apply to CARD-FISH and nanoSIMS images, and are 10 μm (a,b) and 5 μm (c,d). Control A.Carb-3439 aggregates (n=3) incubated with unlabelled chemical substrate exhibited average15N and13C atm % values of 0.35 and 0.54, respectively. Porosity and permeability values of representative samples were empirically measured using core plug analysis to quantify the fluid flow potential through the physical substrates and characterize putative microbial habitats ( Supplementary Table 2 ). Active massive carbonate samples (A.Carb-4588E3 and A.Carb-5152) had permeabilities of 1.7 × 10 −15 to 4.9 × 10 −15 m 2 , while low-activity massive carbonates (L.Carb-5473, L.Carb-5028, L.Carb-2719 and L.Carb-2787; Supplementary Fig. 2g ) were two orders of magnitude less permeable, averaging 1.3 × 10 −17 ±1 × 10 −17 m 2 s.e. Active porous carbonates analogous to chemoherm samples reported in Bahr et al. [19] (for example, A.Carb-5305 and A.Carb-3439; Supplementary Fig. 2e ) were too friable for core plug analysis, but probably exhibit even higher permeabilities given their macroscale vugs and conduits. Petrographic thin sections provide microscopic evidence of less-developed pore-filling aragonite fans and less-dense micritic matrix in active porous carbonates compared with lithified structures from low-activity seep areas ( Supplementary Fig. 3 ). Microbial 16S rRNA gene analysis revealed abundant methane seep-associated archaeal and bacterial phylotypes with an apparent shift in community composition with lower seep activity ( Supplementary Data 1–3 ). Among Archaea, ANME lineages were the predominant sequences recovered at sites within active seep areas, including sediment (92.9%, n =170 total clones), sediment-hosted carbonate nodule (85%; n =113) and exhumed carbonate slab (70.9%; n =206) environments, while a carbonate sample from a region of low methane flux contained a much smaller percentage of ANME representatives (12.9%; n =139; Supplementary Data 1 ). Members of the ANME-1 group comprised nearly all of the recovered ANME sequences within the low-activity seafloor carbonate (83.7%), compared with <40% in active samples (12.7%, 39.6% and 20.6% of ANME sequences in sediment, nodules and carbonates, respectively). The presence of ANME-1 within low-activity carbonate rock was confirmed with FISH, using an ANME-1-specific oligonucleotide probe [32] . Deltaproteobacteria , including representatives closely related to sulphate-reducing genera that associate with ANME in seep environments, accounted for large percentages of the bacterial clones from active sediment (27.3%; 45 sequences) and nodules (53.6%; 75 sequences), but comprised a smaller proportion of recovered sequences within the carbonates from active and low-activity areas (15.2% and 22.7%, respectively, 74 total sequences). Known aerobic methanotrophic sequences were not recovered in 16S rRNA gene bacterial surveys ( Supplementary Data 2 ), but Methylococcales sequences were identified in 454 pyrotag sequencing of the A.Carb-3439 carbonate (14 of n =7,124 reads; Supplementary Data 3 ). Genes encoding particulate methane monooxygenase ( pmoA ), the enzyme responsible for the first step of aerobic methane oxidation, were detected by PCR and sequenced from active seep sediment (A.Sed-3452, 3–6 cm depth horizon) and a carbonate sample recovered off-seep (L.Carb-3414; Genbank accession numbers KF616507 - KF616827 ). Cell aggregates of Archaea and sulphate-reducing deltaproteobacteria were observed by catalysed reporter deposition FISH (CARD-FISH) using the general archaeal probe Arch915 and Desulfosarcina / Desulfococcus ( DSS )-specific probe DSS658 in all carbonates examined, revealing the presence of endolithic microorganisms with intact ribosomes. Quantification of DAPI (4′,6-diamidino-2-phenylindole)-stained cells and cell clusters showed that microbial aggregates within the interior of active carbonates were more abundant and larger, but less densely packed, than sediment- and nodule-hosted aggregates ( Table 1 and Supplementary Fig. 4 ). A ‘pair correlation statistic’ [33] supported this packing density trend, suggesting that cells from sediment-hosted microbial aggregates favoured a shorter intercellular distance (0.59±0.02 μm) than aggregates from nodules, active porous and active massive carbonates (~1 μm). 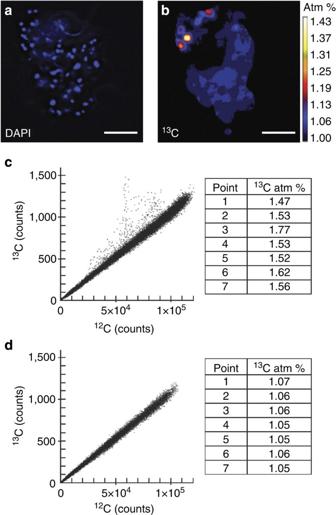Figure 3: Anabolic incorporation of isotopically labelled substrate after brief oxic incubation. (a) DAPI and (b)13C atom % NanoSIMS images of aggregate 27 from sample A.Carb-3439 are shown following a 5-day incubation with13CH4and air headspace. (c) A scatter plot of individual pixels’13C and12C counts from nanoSIMS analysis shows that many pixels skew heavy for the incubated aggregate while (d) none skew away from the mode ratio in a control A.Carb-3439 aggregate incubated without labelled chemical substrates (corresponding control aggregate images not shown). Tables incanddprovide13C atom per cent values for several cell-sized regions of interest acquired from various nanoSIMS cycles during analysis of the experimental and control aggregate, respectively. Scale bar, 5 μm. The vast majority of observed biomass was in aggregate form: microscopic analysis of microorganisms concentrated on 0.22 μm filters showed that <1% of DAPI-stained cells were in single or few-celled arrangements in active rocks, sediments and nodules, while a larger proportion (~10–15%) was observed in low-activity sediment and carbonate rock samples ( Supplementary Table 3 ). Table 1 The average diameter, abundance, biovolume and pair correlation peak of DAPI-stained aggregates across all sample types. Full size table Combining measurements of aggregates’ abundance, size and biovolume within the different habitats surveyed in this study, we calculated that active carbonate habitats had greater aggregate-based microbial abundances per unit dry mass than active methane seep sediment and nodules. Porous carbonates and massive carbonates from active methane seeps hosted 41% and 5% more aggregate-based cells than active seep sediment (per unit mass), respectively, and 143% and 81% more than sediment-hosted carbonate nodules, respectively ( Table 1 ). Methanotrophic metabolic activity To verify whether the carbonate-hosted communities were active in methane oxidation, a 14 CH 4 radiotracer method was used to directly demonstrate net methane consumption by endolithic microorganisms. Methane oxidation was highest in active methane seep sediment (A.Sed-5128, 0–12 cm depth horizon) incubated under anoxic conditions, consuming 193.6±20.4 nmol CH 4 cm −3 per day after a 7-day incubation at 4 °C ( n =3). Porous (A.Carb-5305) and massive (A.Carb-5152) carbonates from active seep sites oxidized methane at rates ~42% and 27% of the sediment AOM rate, or 80.9±9.2 and 52.5±8.0 nmol CH 4 cm −3 per day, respectively. When scaled by relative DAPI-stained aggregate biomass ( Table 1 ), porous carbonates consumed methane at 30% of the rate of active seep-associated sediment per unit biomass and massive carbonates were 26% as active. Sediment and carbonate samples from the lower methane flux sites (L.Sed-5043 and L.Carb-5028) both demonstrated low, but detectable, levels of AOM activity (7.5±1.8 and 11.8±2.0 nmol CH 4 cm −3 per day, respectively). Rates of methane oxidation under oxic conditions were also measured using parallel incubations amended with CH 4 (2.2 mM) and O 2 (420 μM). Aerobic methane oxidation rates were ~31% that of their anaerobic counterparts for both sediments and carbonates among active methane seep samples and 60% among low-activity samples. In all data presented here, rates derived from killed control incubations were subtracted (1.2 and 0.6 nmol CH 4 cm −3 per day for anaerobic-sterilized active sediment and active porous carbonate, respectively; 3.1 and 2.9 nmol CH 4 cm −3 per day for oxic-sterilized active sediment and active porous carbonate, respectively; Fig. 1 ). Figure 1: Methane oxidation rates derived from 14 CH 4 radiotracer experiments. Rates under ( a ) oxic and ( b ) anoxic conditions are shown, using active sediment (A.Sed-5128), low-activity sediment (L.Sed-5043) and intact pieces of active porous carbonate (A.Carb-5305), active massive carbonate (A.Carb-5152) and low-activity massive carbonate (L.Carb-5028) from Hydrate Ridge. Each bar represents nmol methane oxidized at a particular time point, with values from killed control experiments subtracted; error bars show s.e. for triplicate incubations (the 1.9-day aerobic low-activity sediment and 3-day anaerobic active porous carbonate data points represent only one replicate). Full size image To confirm the viability and anabolic activity of carbonate-associated archaea and bacteria, targeted FISH–nanoSIMS analyses were conducted using samples from an active porous carbonate (A.Carb-3439; Supplementary Fig. 2e ), collected from Hydrate Ridge. Following amendment of intact interior pieces of carbonate (~5 cm diameter pieces, ~300 g total mass) with 2 mM 15 NH 4 Cl and 0.44 mM CH 4 (50% 13 CH 4 ) at 4 °C for 27 months, three endolithic archaea and DSS aggregates were identified by CARD-FISH and their 13 C/ 12 C and 15 N/ 14 N ratios measured by nanoSIMS. All three consortia showed maximum levels of 15 N incorporation ranging from 83.3 to 87.9 atom% ( Fig. 2a–c ), demonstrating consistent overall growth rates over an extended incubation period. Carbonate-hosted aggregates had maximum 13 C values of 1.11–1.36 atom% after 27 months, which was approximately double that of the 13 C/ 12 C ratios measured from unlabelled control aggregates (0.48–0.66 atom%; Supplementary Table S4 ). Figure 2: Anabolic incorporation of isotopically labelled substrate by endolithic microbial aggregates. Paired CARD-FISH and nanoSIMS results of samples A.Carb-3439 ( a – c ) and A.Nod-3294 ( d ) are provided. A.Carb-3439 was incubated at 4 °C for 27 months under anoxic conditions with 2 mM 15 NH 4 Cl and 1.48 mM CH 4 (50% 13 CH 4 ); A.Nod-3294 was incubated at 4 °C for 9 months under anoxic conditions with 1 mM 15 NH 4 and 1.12 mM 12 CH 4 . In A.Carb-3439 CARD-FISH images, red signal indicates Arch 915 hybridization and green indicates DSS 658 hybridization; the colours are reversed for A.Nod-3294 hybridizations. 15 N and 13 C atom % nanoSIMS images are derived from 15 N 12 C − / 14 N 12 C − and 13 C − / 12 C − ion count ratios, respectively, and represent mean values from multiple planes of analysis. Scale bars apply to CARD-FISH and nanoSIMS images, and are 10 μm ( a , b ) and 5 μm ( c , d ). Control A.Carb-3439 aggregates ( n =3) incubated with unlabelled chemical substrate exhibited average 15 N and 13 C atm % values of 0.35 and 0.54, respectively. Full size image FISH–nanoSIMS analysis of 15 NH 4 + assimilation by ANME/SRB aggregates recovered from intact sediment-hosted carbonate nodules (~15 mm diameter) also demonstrated significant enrichment after 9 months, reaching 15 N values of 76 atom% ( Fig. 2d ), while aggregates from parallel unlabelled control incubations had 15 N values of ~0.5 atom%. In addition, nanoSIMS analysis of a 5-day shipboard incubation experiment with an intact active carbonate sample (A.Carb-3439, ~10 cm diameter subsample) amended with 0.44 mM CH 4 (50% 13 CH 4 ) and O 2 (air) revealed that half of the DAPI-stained microbial aggregates analysed ( n =10) showed slightly elevated levels of 13 C in biomass relative to the parallel unlabelled controls ( n =3 aggregates; Fig. 3 ). Figure 3: Anabolic incorporation of isotopically labelled substrate after brief oxic incubation. ( a ) DAPI and ( b ) 13 C atom % NanoSIMS images of aggregate 27 from sample A.Carb-3439 are shown following a 5-day incubation with 13 CH 4 and air headspace. ( c ) A scatter plot of individual pixels’ 13 C and 12 C counts from nanoSIMS analysis shows that many pixels skew heavy for the incubated aggregate while ( d ) none skew away from the mode ratio in a control A.Carb-3439 aggregate incubated without labelled chemical substrates (corresponding control aggregate images not shown). Tables in c and d provide 13 C atom per cent values for several cell-sized regions of interest acquired from various nanoSIMS cycles during analysis of the experimental and control aggregate, respectively. Scale bar, 5 μm. Full size image The data presented above demonstrate that methane-derived authigenic carbonates, including sediment-hosted nodules and well-lithified carbonate rocks and pavements at the seabed, host substantial active microbial biomass capable of methane oxidation under both oxic and anoxic conditions. Porosity and permeability heavily influence the microbial habitability of rock-hosted environments by determining both the habitable volume and the dynamics of chemical substrate delivery (CH 4 , SO 4 2− and nutrients) and end-product removal (e.g., H 2 S and HCO 3 − ). The measured permeability values, which indicate connected pore spaces within rock ( Supplementary Table 2 ), ranged over three orders of magnitude. Permeability values of active massive carbonates are within the range of values observed for seep sediments [34] , indicating that fluid flow through the carbonate interior is sufficient to support biological activity. It was not possible to determine the porosity and permeability of active porous carbonates, but their macroscopic vugs and fractures probably confer even higher values; indeed, similar porous structures are reported to harbour localized microbial mats [19] , biomarkers and depleted carbon isotopic signatures [6] in chemoherms. Such enhanced fluid supply is an important environmental variable, particularly in surface-exposed porous carbonates unencumbered by lower-permeability overlying sediment, and may influence microbial aggregate size, abundance and spatial structure. The massive carbonates recovered off-seep from low-activity sites demonstrate much lower permeabilities, likely to be due to the time-integrated accumulation of biologically produced carbonate [13] . Similar permeability decreases occur within modelled mid-ocean ridge basaltic crust, as anhydrite and sulphide precipitation limit fluid flow [35] , and these physical constraints, which could limit methane and nutrient flux, may curtail in situ microbial growth. Active massive carbonates exhibit permeability values similar to those of seafloor basalts, which have been shown to host endolithic chemolithoautotrophic microorganisms [24] . In comparison, permeabilities of massive carbonates from low-activity areas are analogous to those of basalts several hundreds of metres below the seafloor [36] . The organisms we detected in this hydrologic regime may exhibit adaptations to limited chemical substrate delivery; studying these unique ecosystems may provide insight into survival strategies under physical constraints. The methanotrophic communities identified within carbonate rocks appeared to differ across the sampled range of seepage activities and habitat types. In archaeal 16S rRNA gene clone libraries, ANME lineages were decreasingly prominent from active seep sediment (92.9%) to active carbonate nodule (85%), to active seep carbonate (70.9%) habitats; this progressive decrease may point to a physical substrate-based influence on community structure in which additional niches develop in lithified carbonates. The ANME contingent of the carbonate sample from a low-activity site not only comprised a smaller percentage of total archaeal sequences (12.9%) but was also dominated by ANME-1, in contrast to the ANME-2-rich assemblages found at actively venting seeps. ANME-1 archaea may be capable of methanogenesis [37] and have been found to live independently of bacterial partners, indicating that they may not require the close spatial association of syntrophic bacteria [38] . It is possible that ANME-1 in low-activity carbonates adopt multiple configurations, from bacteria-independent monospecific aggregates to ANME-1-deltaproteobacterial consortia. Low-activity carbonates recovered from outside the seep area retained significant microbial biomass in the carbonate interior, much of which appeared to be unrelated to seep-associated microorganisms and suggests a secondary colonization after methane flux wanes. Nonetheless, the occurrence of methanotrophic activity upon the addition of methane indicates the presence and viability of anaerobic and aerobic methane-oxidizing microorganisms, an observation supported by our FISH detection of ANME-DSS aggregates in these samples. Endolithic aggregates recovered from active carbonates were larger and more diffusely packed than those described from active seep sediments ( Table 1 and Supplementary Fig. 4 ), exhibiting mixed or clustered species distributions. When modelling large aggregates (25 μm), Orcutt and Meile [39] found that consortia partners in shell-type aggregates were too distant for electron-carrying intermediates to diffuse out of the archaea-dense inner core at metabolically feasible rates. The observed patchy arrangement of syntrophic partners within large aggregates suggests that their diffusive regimes may be similar to those of smaller aggregates. The diffuse cell packing we observe in endolithic aggregates may represent a transition to a more biofilm-like mode of growth, in which secreted polymeric substances offer a community-wide competitive advantage [40] despite higher localized diffusion coefficients [41] . The rates of AOM measured by 14 CH 4 radiotracer were within the range of previously reported rates from Hydrate Ridge and other seep sites ( Table 2 ). Porous and massive carbonates from active seep sites performed AOM at rates commensurate with active seep sediment [42] , [43] , [44] , while sediment and carbonate rates from off-seep, low-activity areas were similar to those reported from continental shelves [10] , [45] , [46] . Within the comparative context of FISH–nanoSIMS analysis, active porous carbonate-hosted Archaea- DSS aggregates under anoxic conditions display substantial 15 N incorporation compared with aggregates from unlabelled incubations, confirming significant anabolic activity associated with cells residing in carbonate interiors. 15 N-enrichment values were consistent with those of ANME/DSS aggregates measured from 6-month 15 NH 4 + -amended seep sediment incubations [47] and roughly half of those reported in time series analyses by Orphan et al. [48] 13 CH 4 incorporation into AOM biomass has been reported to be ~1% of the total methane oxidized [49] , and thermophilic anaerobic methanotrophic microorganisms have been shown to derive most of their biomass from inorganic carbon sources [50] . Our results were consistent with these observations and the related prediction of substantially lower methane-derived 13 C enrichment than NH 4 + -based 15 N uptake ( Supplementary Table 4 ). 15 NH 4 + uptake was also observed in active nodule-hosted consortia after 9 months ( Fig. 2d ), with enrichment levels suggestive of approximately two or three doublings, similar to estimated growth rates reported from incubations of sediment samples from an active methane seep [47] . Table 2 Comparison of methane oxidation rates. Full size table NanoSIMS analysis of carbonate-hosted communities was suggestive of aerobic methane oxidation potential, although known bacterial methanotrophs were not recovered in 16S rRNA gene clone libraries. Observable 13 C enrichment from AOM requires extended incubations, considering that ANME-SRB consortia have doubling times of several months [49] . Thus, the enrichment observed in our 5-day incubation is probably attributable to aerobic methanotrophs, consistent with the aerobic methane oxidation measured by 14 CH 4 radiotracer experiments. The detection of genes encoding particulate methane monooxygenase in active seep sediment (A.Sed-3452, 3–6 cm depth horizon) and a low-activity carbonate sample (L.Carb-3414), coupled with the observation of Methylococcales sequences from 454 pyrotag sequencing of A.Carb-3439 ( Supplementary Data 3 ), suggests that aerobic methanotrophs are associated with both sediment and exhumed carbonate habitats. However, 16S rRNA gene sequences from known bacterial methanotrophs were not recovered in clone libraries ( n =705 across four sample types; Supplementary Data 2 ), indicating that they may be exceedingly rare members of the community, or that there may be uncharacterized aerobic methanotrophs within the seep carbonate environment. Alternatively, the activity detected under oxic conditions may be due, at least in part, to AOM occurring in anoxic niches, where putative extracellular polymeric substances may confer protection against oxygen exposure. Methane oxidation rates under oxic conditions were ~31±1.2% s.e. that of their anaerobically incubated counterparts for both sediments and carbonates among active methane seep samples and 60±2.8% s.e. among samples from low-activity, seep-adjacent sites. The consistent proportions of aerobic methanotrophic to ANME activity among different sample types, demonstrated by the low s.e., contrasts the samples’ varying microbial community assemblages. These findings suggest that low-abundance microorganisms, both anaerobic and aerobic, maintain viability under quiescent periods of methane flux and are able to initiate activity soon after the introduction of stimulating conditions. It appears that waning methane supply does not necessitate ecosystem shutdown, but rather represents a selective force that presents alternative niches and promotes the successional development or persistence of an endolithic microbial assemblage that retains the capacity for continued methane consumption. The observation of actively metabolizing methanotrophic organisms within carbonate rocks at sites of active and low-activity methane seepage furthers previous studies linking methanotrophic microorganisms with authigenic carbonate formation and shifts the geobiological perception of seep-associated authigenic carbonates. The association of methanotrophic organisms with active porous chemoherms at Hydrate Ridge has been previously postulated [6] , but the associated petrographic, isotopic and microfossil evidence from porous carbonate lithologies (such as that represented by A.Carb-3439 panels in Supplementary Fig. 3 ) stopped short of demonstrating contemporary endolithic activity and net methane consumption. In contrast to such studies of porous chemoherms and carbonate-associated ANME biofilms in the euxinic Black Sea, which cover outer surfaces of carbonate reefs [18] or line centimetre-scale cavities [19] , some of the active AOM assemblages described here persist within pore spaces of highly lithified, low-permeability structures that pave the seafloor and are volumetrically dominant at active and dormant seep sites. We report active and abundant methanotrophic microorganisms not only in porous carbonates at seepage sites with high CH 4 flux, but indeed within carbonates from all investigated seafloor environments, including the abundant low-permeability massive carbonate pavements covering regions of low-seepage activity. These findings suggest that such endolithic communities may be broadly distributed across a wide range of methane- and sulphate-infused carbonates. Endolithic aerobic methanotrophic and ANME communities occupy a previously undescribed niche, replete with distinct physicochemical challenges such as potential nutrient limitation or metabolic product accumulation. There are fundamental similarities in community structure and aggregate morphology between endolithic and sediment-hosted methanotrophic communities, but the distinct parameters of rock-hosted habitats probably promote a unique set of metabolic responses or interspecies spatial relationships, as revealed by our recovery of larger, less-cohesive endolithic aggregates ( Supplementary Fig. 4 ). Understanding the full metabolic repercussions of the endolithic methanotrophic lifestyle—and how it differs from the more familiar sediment-based mode in terms of methane processing or environmental interaction—is a compelling direction of future work. Endolithic methanotrophs within authigenic cold seep mounds may also serve as a useful point of comparison with communities associated with chemically precipitated carbonates at warmer chemolithotrophic habitats such as Lost City. Endolithic methanotrophs likely play an integral role within the larger context of global methanotrophy and methane cycling. Although the extents of both methane seepage and associated authigenic carbonates on a global scale are poorly constrained, targeted studies from select regions indicate that methane seeps and vents are significant contributors to net methane oxidation and are frequently accompanied by substantial carbonate formation [15] , [27] . Along the Costa Rica margin, multibeam bathymetry, side-scan sonar imagery, remotely operated vehicle observations and sampling revealed more than 100 previously unknown seep sites, typified by authigenic carbonate mounds rising up to 100 m above the seafloor [23] . At better-characterized sites, published side-scan sonar results, seafloor photographic images and descriptions of seep sites indicate that ~46% of active methane seep sites at the seabed are paved by authigenic carbonates [4] , [5] , [6] (surveyed sites include Hydrate Ridge, the Costa Rica margin, Santa Monica Basin and the Chilean subduction zone). Assuming methanotrophy at active sites that would otherwise occur in overlying sediment takes place endolithically, we estimate that endolithic AOM in surface-exposed carbonates may account for 12.5 (using massive carbonate rates) to 19.2% (using porous carbonate rates) of the overall methane consumption estimated to take place at active seeps. The endolithic contribution to AOM at low-activity settings and adjacent marine sediment sites is more difficult to quantify. The carbonate samples collected for this study were, by necessity, from exhumed seafloor carbonate pavements, and the extent to which our findings translate to deeper carbonate lenses and platforms requires targeted study. Authigenic carbonates account for the vast majority of mound volume at methane seep complexes: 85.7% at the Costa Rica margin [4] , 99.8% at Hydrate Ridge South Pinnacle and SE Knoll [6] , 99.2% at Chilean seeps [5] and, in regions such as the Florida escarpment, carbonates can pave extensive areas of the seafloor [51] . The high permeability values measured from carbonates at actively venting sites and the emergence of methane-rich fluids above carbonate pavements [52] imply that large carbonate mounds (10 to ~100-m tall) are supplied with abundant methane. Sulphate supply within the carbonate interior may be enhanced by downward fluid circulation, which has been attributed to tidal forcing and/or negative pressure generated by focused fluid discharge [34] , and hydrologic recharge of carbonate masses, previously suggested at the base of methane seep sites including Hydrate Ridge [6] and the Florida Escarpment [51] . With extensive methane and sulphate perfusion of mound carbonates [6] , [34] , [51] , and the recognition that sulphate concentration far below that of ambient seawater can sustain AOM [53] , the potential for endolithic methanotrophy is substantial and may exceed that of surface-associated seep sediments. Hidden sources of endolithic AOM, where either methane availability and/or carbonates have no seafloor surface expression, could further enhance the global contribution of carbonate-hosted communities to methane budgets. Thin carbonate crusts may cut off methane supply to overlying sediments within hundreds of years [54] : this self-sealing effect limits methanotrophy in the upper sediment column but may increase methane concentrations in the underlying carbonate layers [55] and sustain AOM activity, contingent on electron acceptor availability. The recognition of seep-associated carbonates as active and dynamic habitats across a range of geochemical conditions also challenges the treatment of such structures as passive recorders of historical methane seepage. The persistence of actively metabolizing communities in seafloor mound structures makes the deconvolution of modern and fossil microbial assemblages difficult without phylogenetically linked isotopic tracer incubation studies or well-constrained biomarker isotopic relationships. However, any perturbation, including methane-perfused incubations, may stimulate dormant microbial lineages and thus erroneously characterize the metabolic activity and relative abundances of in situ microbial constituents. The extent to which microbial communities in low-activity carbonates are diagnostic of previous seep activity and the rate of community succession between active and inactive seep areas has ramifications for the interpretation of biomarker analysis in ancient seeps [56] . Biomarkers within ancient seep structures [57] are thus time-integrated reflections of a range of physicochemical environments, probably weighted toward particularly productive or recent regimes, and tempered by remineralization, succession and competition among microbial communities. The demonstration of abundant, active methanotrophic microorganisms within authigenic methane seep-associated carbonates reveals a dynamic ecosystem able to adapt to changing environmental conditions and methane fluxes. Given the broad distribution of methane- and sulphate-infused carbonates at and below the seafloor, carbonate-hosted methanotrophy probably represents a globally relevant sink for methane. The discovery of substantial methane consumption by these carbonate-associated microbial communities also marks an important step in our understanding of the extent of viable habitats for anaerobic methanotrophs and associated methane turnover within the marine environment. Sample collection and characterization Samples for the study of endolithic AOM were collected from three convergent boundary cold seep sites: an erosional subduction zone near Costa Rica (Mound 12, 1,000 m depth; 8°55.8′N, 84°18.8′W), Eel River Basin (Northern Ridge, 525 m; 40°48.70′N, 124°36.68′W) and an accretionary prism at Hydrate Ridge, Oregon (Hydrate Ridge South, 800 m; 44°34.09′N, 125°09.14′W and SE Knoll, 620 m; 44°26.99′N, 125°01.97′W). These sites have been previously established as areas of active methane seepage and sediment-based AOM at which methane from seep structures enters the water column at concentrations ranging from 100 nM (Costa Rica) [58] and 200 nM (Eel River Basin) [59] up to 4,400 nM (Hydrate Ridge) [60] . Authigenic carbonates have been shown to adsorb methane and create localized sites of heightened concentrations [61] , and pore water geochemical measurements from selected sediment push cores confirm elevated methane levels and reveal signs of AOM metabolism (pore water extrusion and geochemical analyses from push core sediments were conducted following protocols outlined in Orphan et al. [62] ). For example, sediment porewater measurements associated with the Eel River Basin seep (6–9 cm below seafloor) from which A.Nod-2688 was collected exhibited high levels of sulphide (8.5 mM), depleted sulphate (19.2 mM), and elevated methane (950 μM) and dissolved inorganic carbon (23 mM) with a δ 13 C DIC that is highly negative (−36.1‰), indicative of active methane oxidation. More limited geochemical measurements associated with the Costa Rica methane seep sample from which A.Nod-3294 was recovered were also consistent with active seepage, with pore waters containing 1.23 mM CH 4 , while the Hydrate Ridge seep sediments from which A.Nod-2518 was obtained contained 2.74 mM CH 4 and a δ 13 C DIC of −38.64‰. Sediments, nodules and carbonates were sampled with the DSV Alvin during R/V Atlantis legs AT-15-11 (Hydrate Ridge and Eel River Basin, September–October 2006), AT-15-44 (Costa Rica, February 2009), AT-15-59 (Costa Rica, January 2010), AT-15-68 (Hydrate Ridge, August 2010) and with ROV Jason during AT-18-10 (Hydrate Ridge, September 2011). Samples included 6 sediment cores, 4 sediment-entrained nodules and 14 carbonates naturally exposed at the seafloor; all samples were kept at ambient bottom water temperatures (~4 °C) during recovery. Supplementary Table 1 provides a more detailed accounting of the origin, activity and degree of lithification of all samples referenced herein via serial number, and Supplementary Fig. 2 presents images of representative samples. Average δ 13 C carbonate values from both active (A.Carb-2840: −48.3‰; A.Carb-2871: −27.5‰; A.Carb-3439: −38.5‰) and low-activity carbonates (L.Carb-2874: −28.5‰; L.Carb-3414: −38.2‰) indicate the incorporation of 13 C-depleted, methane-derived carbon. The ‘active’ designation refers to sites where methane seepage was manifested by seafloor ecosystems known to be fueled by subsurface methane (mussel beds, tubeworm bushes, clam beds, provannid snails and bacterial mats) or methane bubble ebullition ( Supplementary Fig. 1a,b ). Authigenic carbonate precipitates, whose calcium carbonate mineralogy was confirmed with X-ray diffraction, form loosely consolidated protoliths heretofore referred to as ‘nodules’ within active sediments. With further precipitation and compaction in a methane-perfused regime, larger carbonate rocks (or ‘active carbonates’) form, which can be uplifted and exhumed, generating extensive pavements around methane seeps [62] , [63] . The term ‘low activity’ references sampling sites that did not exhibit any clear signs of methane seepage or chemosynthetic communities, although methane supply cannot be entirely ruled out, as subsurface advective flow can shift with time [43] , [64] . Low-activity sites were comparatively barren, yet δ 13 C carbonate values and the carbonate mineralogy of such samples suggest that they formed in ‘active’ seep settings. In all experiments involving carbonates, interior portions (>5 cm from the surface) were used in to ensure that properties exhibited were representative of bulk rock material and not a reflection of surface-based adherent cells or entrained material. At seep-associated mounds, carbonate rocks form extensive pavements and are often overlaid by thin veneers of sediment and/or microbial mats ( Supplementary Fig. 1c,d ). The thickest layers of sediment associated with active seep areas often occur between carbonate blocks in depressions that may have formed as a result of localized faulting. At low-activity sites, carbonate surface expression is less pronounced, although deposits of unsedimented carbonates are apparent ( Supplementary Fig. 1e,f ). X-ray diffraction Two samples of sediment (A.Sed-3098, A.Sed-3452), nodule (A.Nod-3099, A.Nod-3294), active carbonate exterior (A.Carb-4588E3, A.Carb-5305), active carbonate interior (A.Carb-4588E3, A.Carb-5305), low-activity carbonate exterior (L.Carb-2874, L.Carb-3604) and low-activity carbonate interior (L.Carb-2874, L.Carb-3604) were powdered with a sterilized ceramic mortar and pestle. The relative intensity of X-ray reflections as a function of beam incidence angle was measured with a Phillips X’Pert Multi Purpose X-Ray Diffractometer. SiO 2 was used as a standard, and best-fit analyses (with peak-shifting permitted) were conducted with the X’Pert HighScore software and its library of diffractograms. Porosity and permeability Porosity and permeability tests were conducted by Weatherford Laboratories (Humble, TX) on 2.54-cm diameter core plugs between 5 and 7.5 cm in length. Porosity was determined with Boyle’s Law Single Cell method, a non-destructive technique that quantifies porosity directly without the need for disaggregation. Permeability was calculated using Darcy’s Law incorporating measured flow rates through the core plug under a range of pressures. Details on porosity and permeability methodology can be found in the American Petroleum Institute’s Recommended Practices for Core Analysis [65] . Petrographic analysis Five thin sections—representing three active (A.Carb-2840, A.Carb-3439 and A.Carb-3460) and two low-activity carbonates (L.Carb-2874, and L.Carb-3414)—were prepared by Spectrum Petrographics (Vancouver, WA) with blue epoxy embedding and visualized across a range of magnifications with a Leica DM 2500P microscope and Nikon DXM 1200F camera. All thin sections were prepared with a thickness of 30 μm. Phylogenetic analysis To acquire 16S rRNA gene sequences, the following workflow was performed for active sediment (sample A.Sed-3730), carbonate nodule (A.Nod-2518), active carbonate (A.Carb-3439) and low-activity carbonate (L.Carb-3604) samples. DNA was extracted from ~0.5 g of material using the UltraClean Soil DNA isolation kit (Mo Bio Laboratories, Carlsbad, CA). Bacterial and archaeal 16S rRNA genes were amplified in separate PCR reactions as described in the Supplementary Methods . Cleaned, amplified DNA product was cloned into chemically competent E. coli with the TOPO TA Cloning Kit (Invitrogen, Carlsbad, CA). Restriction fragment length polymorphism was performed for bacterial sequences using Hae III and Sau 96I enzymes, and for archaeal sequences using Rsa I and Hae III enzymes; all enzymes were acquired from NEB (Ipswich, MA) and one or two representatives of each unique restriction digest pattern were sequenced by Laragen, Inc. (Culver City, CA). Resulting sequences were aligned, checked for chimeras and plotted as described in the Supplementary Methods . 454 Pyrotag sequencing was performed using the Roche 454 GS-FLX Titanium platform (Roche Diagnostics, Castle Hill, NSW, Australia) at the Australian Centre for Ecogenomics. See Supplementary Methods for details on PCR conditions and amplicon processing. Cell visualization On recovery from the seafloor, carbonate and sediment samples for microscopy analysis were fixed in 2% formaldehyde and stored at 4 °C overnight; the next day, the formaldehyde was washed from the samples with sterile PBS buffer and then transferred into 100% ethanol and stored at −80 °C. In the case of carbonate rocks, interior portions were isolated for analysis by sterile mortar and pestle and sterile razor blade manipulation to minimize the role of surface-based communities. This method of mechanical separation was replicated on sediments; resulting samples, when compared with unprocessed sediment samples, confirmed that the diffuse aggregate morphology, cell abundance and aggregate size found in carbonate samples are not artefacts of mortar and pestle treatment. Aggregate counts were performed using CARD-FISH and DAPI staining on 3-μm polycarbonate filters. To examine the proportion of single cells, sonicated sample material (sonicated on ice 3 × 10 s at 8 W; Branson sonifier 150) was concentrated on a 0.22-μm polycarbonate filter and stained with DAPI. Twenty-five fields of view were surveyed to determine the proportion of cells present as single cells. Cell and aggregate counts were normalized per unit dry mass for all sample types. Samples for CARD-FISH were prepared as follows. To concentrate cell aggregates, a percoll density separation was performed according to Orphan et al. [38] Fixed, crushed sample was permeabilized by mixing 60 μl sample with 1,290 μl TE (pH 9) and heated for 3 min at 60 °C. The sample tubes were put on ice for 5 min; 4.5 μl of 30% H 2 O 2 was then added (to deactivate peroxidase) and incubated at room temperature for 10 min. Tubes were put back on ice and 150 μl sodium pyrophosphate were introduced. Sample mixtures were sonicated on ice three times at 8 W for 10 s each time and applied to the density gradient vials. The vials were then centrifuged at 4,800 r.p.m. for 15 min at 4 °C. The supernatant was filtered through a 3-μm filter, which was then rinsed with 2 ml PBS and dehydrated with 2 ml 1:1 ethanol:PBS. For samples intended for nanoSIMS analysis, percoll-prepared aggregates were concentrated onto a 3-μm-pore-sized polycarbonate filter and inverted onto an indium tin oxide-coated glass slide to transfer biomass as described in Orphan et al. [38] For samples only visualized with DAPI, the above protocol was followed with the exception of the permeabilization and peroxidase deactivation steps. CARD-FISH reactions on slides and filters were performed as in Dekas et al. [47] (see Supplementary Methods for additional details.). All visualizations and cell counts described above were conducted with epifluorescence microscopy using a 60 × objective lens (Olympus BX51 microscope, Olympus, Melville, NY). Aggregate spatial analysis Aggregate architecture was examined with the DAIME image analysis and three-dimensional visualization programme [33] . By recognizing fluorescent biomass within manually set aggregate boundaries throughout a z -stack of images, DAIME is able to calculate biovolume and the pair correlation function. Biovolume is determined by dividing the three-dimensional integrated volume of cells by the overall aggregate volume. To derive the pair correlation function, the programme rasters across the entire aggregate, deploying dipole lines of varying lengths in all directions at each pixel. If each end of the dipole contacts a distinct object (that is, a cell), a hit is recorded at that dipole length. By ratioing the dipole hits to total dipoles as a function of dipole length and normalizing by cell density, the pair correlation statistic is obtained; its peak value corresponds to the most favoured cell–cell distance. Biovolume and pair correlation values were obtained from five representative aggregates from each environment; cell sizes were consistent for all samples. 14 CH 4 rate measurements Methane oxidation rates at two times points were measured for each of seven samples: A.Sed-5128, A.Carb-5305, A.Carb-5152, L.Sed-5043, L.Carb-5028 and sterilized control aliquots of A.Sed-5128 and A.Carb-5305. All incubations contained 10 ml physical substrate (compressed sediment or carbonate rock) and 20 ml filtered Hydrate Ridge bottom water. Carbonate rock samples were fragmented to fit through the 28-mm diameter bottle opening (SVG-50 gaschro vials, Nichiden Riku Glass Co., Kobe, Japan); pieces were kept as large as possible to minimize the increase in surface area-to-volume ratio and maintain conditions as representative of the in situ environment as possible. Following several minutes of flushing with N 2 (g), 60 ml of gas was injected into the 30-ml headspace, generating a pressure of ~2 atm. Anaerobic incubation headspace was 100% CH 4 ; aerobic incubation headspace was 30 ml CH 4 , 20 ml N 2 and 10 ml O 2 . All incubation set-up before gas flushing and injection took place in an anaerobic chamber. Triplicate incubations for each sample/headspace combination (which represented subsamples of the sample type population) were set up for each of two time points, with the exception of sterilized controls, which were sampled only at the second time point. In total, 72 incubations were prepared and maintained with a CH 4 headspace at 4 °C for 2 weeks before radiolabel addition to establish consistent environmental conditions. Rates of methane oxidation were measured following the methods of Treude et al. [66] ; details are provided in the Supplementary Methods . The rate of methane oxidation can then be determined by the equation in which 14 CH 4 is the combusted unreacted radiolabelled methane, 14 CO 2 represents the quantity of acidified oxidation product, CH 4 signifies the initial quantity of methane in the experiment, v is the volume of sediment or carbonate rock and t is the time over which the incubation was active. Methane oxidation rates from control incubations were attributed to abiotic activity, and these values (3.1 nmol CH 4 cm −3 per day for aerobic sediment, 2.9 nmol CH 4 cm −3 per day for aerobic carbonate, 1.2 nmol CH 4 cm −3 per day for anaerobic sediment and 0.6 nmol CH 4 cm −3 per day for anaerobic carbonate) were subtracted from experimental treatments to yield the final biological oxidation rate values. NanoSIMS measurements Target aggregates from CARD-FISH analysis were mapped on indium tin oxide-coated glass squares using both epifluorescence and transmitted light microscopy with a DeltaVision RT (Applied Precision Inc., WA) according to Dekas et al. [47] The Cameca nanoSIMS 50L was used to collect high-resolution data on isotopic uptake in nodule and carbonate rock incubations; 15 N 12 C − , 14 N 12 C − , 13 C − and 12 C − ions were collected. For our analyses, a 2.5-pA caesium beam with a spot size of 100–200 nm was used. The beam rastered over areas dependent on the size of the aggregates selected (generally between 5 and 20 μm) with a 256 × 256 pixel resolution, a dwell time of 5–10 ms per pixel and a resolving power of ~5,000. Multiple frames, each lasting ~30 min, were taken per aggregate (between 5 and 60 frames), as the beam sputtered away layers of material. NanoSIMS images were processed with L’image (developed by L. Nittler, Carnegie Institution of Washington, Washington D.C.). Each set of frames was corrected for drift and detector dead time. Discrete regions of interest were drawn manually on the ion images based on the corresponding CARD-FISH data; isotope ratios were subsequently calculated for these regions. The following samples were analysed: A.Nod-3294 incubated for 9 months amended with 1 mM 15 NH 4 Cl and an unlabelled methane headspace in a 125 ml vial; A.Carb-3439 incubated under air for 5 days in an air-tight mylar bag (~800 ml) with the addition of 0.74 mM 12 CH 4 and 0.74 mM 13 CH 4 ; A.Carb-3439 incubated for 27 months under anoxic conditions with 2 mM 15 NH 4 Cl, 0.74 mM 12 CH 4 and 0.74 mM 13 CH 4 . Parallel incubations of aliquots treated with unlabelled NH 4 Cl and CH 4 chemical substrates served as controls. All incubations were set up shipboard, within hours of sample recovery from the seafloor (after several minutes of Ar sparging in the case of anoxic experiments). The extended incubations, during which methane was not replenished and the water was not flushed, probably influenced the composition and activity of resident microbial communities as the methane-sourced carbon may transition through multiple pools before analysis. However, when dealing with organisms that grow at such low rates (doubling times in excess of a month), such long anabolism-based incubations are necessary. Understanding these limitations, growth rates derived from nanoSIMS data should be viewed as conservative estimates; the primary utility of the method is to definitively demonstrate anabolic activity through the isotopic enrichment of cell material. Sterilized control incubations were not measured by nanoSIMS analysis, but isotopic enrichment was exclusively observed in association with Archaea-SRB aggregates (as established by CARD-FISH), indicating that abiotic isotopic incorporation was not statistically significant. All incubations were conducted in anoxic filtered Hydrate Ridge bottom water at 4 °C. Clostridia spores with known 13 C/ 12 C and 15 N/ 14 N ratios (measured by conventional elemental analyzer-isotope ratio mass spectrometer, EA-IRMS) were used as a standard and measured before and after sample analysis to track instrumental mass fractionation and drift over the course of the nanoSIMS analysis session. The 13 C and 15 N ratios of Clostridia spores analyses bracketing our samples were consistent throughout the run. The 13 C/ 12 C ratios of the unlabelled control archaeal— DSS aggregates were below natural abundance and can be attributed to the incorporation of 13 C-depleted carbon from the methane-seep environment [48] , instrument-associated fractionation [67] or biological matrix effects [68] . Although the accuracy of the natural abundance δ 13 C values for aggregates in control incubations is poorly constrained, these samples serve as a comparative reference for our 13 CH 4 amended samples. pMMO analysis Particulate methane monooxygenase genes (pmoAC) were amplified from extracted DNA using the MISA PCR assay as described previously by Tavormina et al. [69] Products were cloned into pSMARTGC LK-kan (Lucigen Corp., Middleton, WI) following the manufacturer’s guidelines. Forty-two colonies from sample L.Carb-3414 and 46 from A.Sed-3452 were picked and amplified with SL1f (5′-CAG TCC AGT TAC GCT GGA GTC-3′) and SR2r (5′-GGT CAG GTA TGA TTT AAA TGG TCA GT-3′); the product DNA was digested with restriction enzyme Rsa I. Representative restriction fragment patterns were selected and the corresponding DNA was sequenced by Laragen, Inc. (Culver City, CA). Resulting sequences were processed and aligned using the Sequencher software and chimeras were removed. Pmo sequences recovered in this study have been submitted to Genbank under accession numbers KF616507-KF616827. Estimates of carbonate volume and aerial cover The relative volumes of carbonate rock and overlying sediment at several cold seep sites were estimated by compiling side-scan sonar data, photographs and descriptions from previously published studies. The proportion of mound volumes attributable to carbonate rock was determined by side-scan sonar images of vent fields, in which high backscatter is interpreted as carbonate rock and from which depths of carbonate extent can be estimated [4] . The average thickness of the overlying sediment layer is known from published reports [4] , [5] , [6] , allowing for the calculation of the proportion of active methane seep mound volume occupied by potentially habitable carbonate rock. (This calculation approach fails to detect carbonate nodules within sediment, thereby minimally underestimating the volume of potentially habitable endolithic habitat.) The estimate of actively seeping surface area covered by carbonate rock is derived from side-scan sonar surface expression data and schematic maps based on extensive in situ observation [4] , [5] , [6] . Accession codes: 16S rRNA gene sequences have been deposited in the Genbank database under accession codes KF616507-KF616827 and KM356196-KM356250. 454 sequences were submitted to the National Centre for Biotechnology Information Sequence Read Archive under experiment ID SRX681843, Run SRR1552592. How to cite this article: Marlow, J. J. et al. Carbonate-hosted methanotrophy represents an unrecognized methane sink in the deep sea. Nat. Commun. 5:5094 doi: 10.1038/ncomms6094 (2014).